Active JNK-dependent secretion ofDrosophilaTyrosyl-tRNA synthetase by loser cells recruits haemocytes during cell competition Cell competition is a process by which the slow dividing cells (losers) are recognized and eliminated from growing tissues. Loser cells are extruded from the epithelium and engulfed by the haemocytes, the Drosophila macrophages. However, how macrophages identify the dying loser cells is unclear. Here we show that apoptotic loser cells secrete Tyrosyl-tRNA synthetase (TyrRS), which is best known as a core component of the translational machinery. Secreted TyrRS is cleaved by matrix metalloproteinases generating MiniTyr and EMAP fragments. EMAP acts as a guiding cue for macrophage migration in the Drosophila larvae, as it attracts the haemocytes to the apoptotic loser cells. JNK signalling and Kish , a component of the secretory pathway, are autonomously required for the active secretion of TyrRS by the loser cells. Altogether, this mechanism guarantees effective removal of unfit cells from the growing tissue. Cells of multicellular animals often compete for extracellular factors that promote their own survival [1] . These factors are traditionally called ‘trophic factors’ and are often released in limiting amounts, supporting the survival of only a fraction of the cells [1] , [2] . In Drosophila , there is a similar process known as cell competition [3] , whereby suboptimal cells are competed out for survival factors and eliminated by apoptosis [4] . Cell competition therefore shares many features with trophic theories, and withdrawal of survival factors is an important event in the elimination of unfit cells not only in Drosophila but also in mammals [5] , [6] . However, it is worth mentioning that recent work in Drosophila suggest that trophic theories may be too simplistic to explain cell selection, because there are mechanisms that allow cells to compare their fitness directly [7] , [8] . Here we focus on the last steps of this cell selection process, when ‘unfit cells’ that did not obtain enough survival factors are excluded from the tissue and engulfed by other cells [9] , [10] , [11] , [12] . In particular, we address the question whether the chemotactic signals originated from the dying cells direct their own engulfment. We have previously described that a significant number of circulating haemocytes reaches the sites where cell competition is taking place [10] , [13] , [14] . To further analyse this recruitment, we studied whether it was active, that is, mediated by chemotactic signals secreted by dying cells, or a passive process. In doing so, we discovered that Drosophila melanogaster Tyrosyl-transfer RNA (tRNA) synthetase, TyrRS, acts as a haemocyte attractant towards dying cells. Aminoacyl-tRNA (AARS) synthases are a group of 20 enzymes, one for each essential amino acid. They catalyse the first step of protein synthesis by binding the specific amino acid with its cognate tRNA. However, during evolution the AARS have acquired new functional domains enabling them to perform activities other than their canonical function [15] , [16] . Thus far, the AARS have been implicated in processes such as angiogenesis, apoptosis and cellular growth [17] , [18] , [19] . The Tyrosyl-tRNA synthetase (TyrRS) possesses the endothelial monocyte-activating polypeptide II (EMAPII) domain that is conserved from insects to humans [20] , [21] , [22] , [23] . Mutations within this element do not alter the canonical function of TyrRS, suggesting that this domain might be implicated in other activities such as angiogenesis [19] , [24] as well as in leukocyte and macrophage recruitment [25] . Mutations in these regions have been associated with neurodegenerative diseases, such as dominant intermediate Charcot–Marie–Tooth neuropathy [20] , which has been modelled in D. melanogaster [21] . Little is known about the molecular mechanisms that drive haemocytes recruitment during cell competition. A better insight into this process may help to understand how multicellular organisms eliminate apoptotic cells. In this study, we show that loser (dying) cells secrete TyrRS, a core component of the translation machinery, through a mechanism that requires the JNK pathway and the secretory regulators Kish and gryzun . Once released TyrRS is cleaved by matrix metalloproteinases (Mmp) in a proteolytic process. The extracellular TyrRS is then capable of activating PI3K in haemocytes acting as a chemoattractant. Thus, we report that apoptotic cells release a signal that recruits haemocytes that in turn engulf the dead cells. TyrRS is secreted by loser cells during cell competition We have shown that Drosophila haemocytes are recruited towards the basal regions where cell competition is taking place to remove apoptotic corpses [10] . To further investigate this recruitment, we searched for molecules that could mediate the chemotactic response during cell competition. To this end, we searched for candidates in a previously described cell competition gene expression microarray [7] . Among the genes that changed their expression profile during cell competition, we found that CG4561 (TyrRS) significantly increased its transcription levels ( Fig. 1a ), reaching maximum expression 24 h after clone induction (ACI) (values are normalized to basal levels of expression, before cell competition is induced, t 0 ). 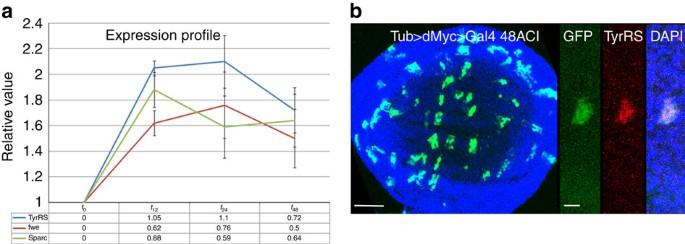Figure 1:TyrRSexpression in loser cells during super-competition. (a)Tyrosyl-tRNA synthetase(TyrRS),flower(fwe) andSparctranscription profiles at different time points (yaxis:t0−t48) after clone induction during cell competition. Average data from triplicates. STD is represented. (b) Staining of endogenous TyrRS (red) in clones ofwtloser cells (green, GFP) under cell competition in wing imaginal discs 48 h after clone induction (ACI). Magnification of a loser cells clone with TyrRS upregulation. Scale bars, 50; 10 μm. Figure 1: TyrRS expression in loser cells during super-competition. ( a ) Tyrosyl-tRNA synthetase (TyrRS), flower (fwe) and Sparc transcription profiles at different time points ( y axis: t 0 − t 48 ) after clone induction during cell competition. Average data from triplicates. STD is represented. ( b ) Staining of endogenous TyrRS (red) in clones of wt loser cells (green, GFP) under cell competition in wing imaginal discs 48 h after clone induction (ACI). Magnification of a loser cells clone with TyrRS upregulation. Scale bars, 50; 10 μm. Full size image Human TyrRS was previously shown to be secreted from human apoptotic cells under serum deprivation and then cleaved into fragments with chemotactic activities [25] . However, no other TyrRS outside humans has been described as a chemoattractant. This raises the question whether this non-canonical function of human TyrRS is conserved in other organisms. To determine whether loser or winner cells upregulate and secrete TyrRS, we generated tub>gal4 wild-type ( wt ) loser cells (green, green fluorescent protein (GFP)) in a tub>dmyc background. In this scenario, the apoptotic loser cells are extruded basally from the epithelium, followed by the haemocyte recruitment to eliminate cell debris [10] . We detected TyrRS upregulation in loser cells by immunostaining ( Fig. 1b ). Furthermore, extracellular immunostaining detected endogenous TyrRS on non-permeabilized wing discs [22] . Extracellular staining revealed the presence of external TyrRS next to loser cells within wing imaginal discs 24 h after induction of super-competition ( Fig. 2a,b,e ), but not in the absence of super-competition ( Fig. 2c,d ). Importantly, TyrRS was also visualized further away from loser cells, suggesting diffusion of secreted TyRS. 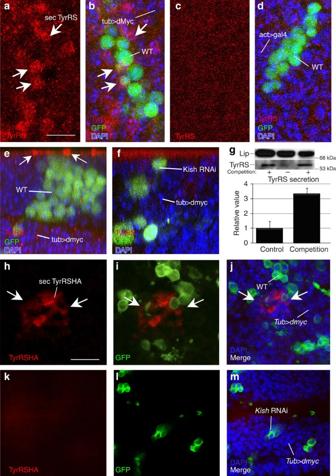Figure 2: TyrRS extracellular staining and haemolymph secretion. (a–d) Extracellular staining of endogenous TyrRS (red) in clones ofwtloser cells (green, GFP) under cell competition in wing imaginal discs (a,b) or without cell competition (c,d). (e,f) Z-section of wing imaginal discs with loser cells (GFP) under cell competition, endogenous TyrRS extracellular staining (red) in clones under cell competition in wing imaginal discs (e) or withKishRNAi co-expression (f). (g) Western blot of Lipophorin (loading control) and endogenous TyrRS in haemolymph of larvae with or without cell competition (48 ACI) and quantification of three independent experiments normalized by loading control (Lipophorin). The difference is statistically significant,T-testP<0.05. (h–j) Extracellular staining of secreted TyrRS (red, anti-HA staining) inwtloser cells (green, CD8-GFP) expressingUAS-TyrRS-HA. Extracellular secretion ofUAS-TyrRS-HAis lost whenKishRNAi is co-expressed (k–m). Scale bar, 10 μm. Figure 2: TyrRS extracellular staining and haemolymph secretion. ( a – d ) Extracellular staining of endogenous TyrRS (red) in clones of wt loser cells (green, GFP) under cell competition in wing imaginal discs ( a , b ) or without cell competition ( c , d ). ( e , f ) Z-section of wing imaginal discs with loser cells (GFP) under cell competition, endogenous TyrRS extracellular staining (red) in clones under cell competition in wing imaginal discs ( e ) or with Kish RNAi co-expression ( f ). ( g ) Western blot of Lipophorin (loading control) and endogenous TyrRS in haemolymph of larvae with or without cell competition (48 ACI) and quantification of three independent experiments normalized by loading control (Lipophorin). The difference is statistically significant, T -test P <0.05. ( h – j ) Extracellular staining of secreted TyrRS (red, anti-HA staining) in wt loser cells (green, CD8-GFP) expressing UAS-TyrRS-HA . Extracellular secretion of UAS-TyrRS-HA is lost when Kish RNAi is co-expressed ( k – m ). Scale bar, 10 μm. Full size image Kish regulates TyrRS secretion during cell competition Using the same assay where wt loser cells were confronted with dMyc-overexpressing super-competitors, we asked whether TyrRS secretion depends on known components of the Drosophila secretory pathway, such as Kish [23] . To this end, we performed an RNA interference (RNAi)-mediated knockdown of kish expression in GFP-labelled loser cells. Staining for extracellular TyrRS ( Fig. 2e,f Z-section) showed that Kish silencing prevented secretion of TyrRS during cell competition ( Fig. 2f Z-section). To exclude the possibility that Kish RNAi affects cell survival or proliferation, we generated WT clones expressing either kish-specific RNAi (marked by GFP expression) or LacZ in a background without cell competition. No differences were observed between the clones 48 h ACI ( Supplementary Fig. 2A–D ). Next, to determine the TyrRS baseline levels in the haemolymph, we compared TyrRS levels in the haemolymph extracted 48 h after induction of super-competition with a no-competition situation by western blot, using an-anti-TyrRS antibody (Covalab) ( Supplementary Video 1 ; Supplementary Fig. 1 ). Three independent experiments were performed and TyrRS levels were quantified and normalized to total protein (Bradford) and anti-Lipophorin [26] amounts ( Fig. 2g ). Of note, higher levels of secreted TyrRS were detected in samples from larvae where cell competition was induced compared with samples from larvae with non-competition clones. To test whether TyrRS was secreted by loser cells, we performed extracellular immunostaining in non-permeabilized wing discs [22] , where WT loser cells overexpressing an HA (haemagglutinin)-tagged version of TyrRS were confronted with dMyc-overexpressing super-competitors (see Methods). Extracellular staining of the HA-tag revealed the presence of extracellular TyrRS in the close proximity to loser cells ( Fig. 2h–j ). Again, the TyrRS secretion was prevented by an RNAi-mediated knockdown of two components of the secretory pathway, Kish and gryzun [23] , in loser cells ( Fig. 2k–m ; Supplementary Fig. 2E–G ). Altogether, these results indicate that TyRS secretion occurs through known components of the secretory machinery, suggesting that it is a regulated process. TyrRS secretion by loser cells is JNK- and kish dependent To test whether TyrRS is as a haemocyte chemoattractant, we first determined whether it was secreted and cleaved by serum-deprived cells, as it has been described in human cells [25] . Drosophila S2 cells were transfected with HA-tagged TyrRS and cultured without serum. Supernatant and cellular fractions were harvested 6 and 24 h after transfection, protein concentration was quantified by the Bradford assay and analysed by western blot. Anti-HA staining revealed comparable expression levels of TyrRS-HA and the presence of secreted TyrRS-HA in the supernatant 24 h after serum deprivation ( Fig. 3a ); however, we could not detect any cleavage of TyrRS-HA, whereas different fragments were observed when larvae haemolymph was analysed (see below). Blots were probed with anti-tubulin antibody to exclude cellular contamination. To rule out the possibility that TyrRS was released by dying cells, we stained cells cultured with or without serum with a green fluorescent dye that marks dead cells with compromised plasma membrane permeability (Sytox Green, Life Technologies) [27] 24 h after transfection with TyrRS-HA ( Fig. 3b–d ). The total number of dead cells was the same under both conditions. As others have reported that S2 cells undergo apoptosis 24 h after serum deprivation [28] , we repeated this experiment using a different lot of fetal bovine serum and cell media. However, contrary to published data, we detected cell death 36 h after serum deprivation ( Fig. 3b–d ). This result indicates that the presence of TyrRS in the conditioned media upon 24 h of serum deprivation is not caused by cell death. 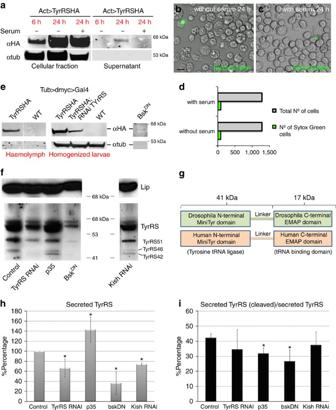Figure 3: Loser cells secrete TyrRS under serum deprivation and during cell competition. (a) Western blot of cellular fraction and supernatant ofDrosophilaS2 cells transfected withTyrRS-HA-tagged (C terminus). Cells are cultured with (+) or without (−) serum, as indicated. Anti-HA is used to detectTyrRS-HAexpression and anti-tubulin is used as a negative control. (b,c) Microscopy images of culturedDrosophilaS2 cells with and without serum at 24 h. Sytox Green is used as a marker of cell death. Scale bar, 25 μm. (d) Quantifications of total number of cells and dead cells. (e, left panel) Western blot of haemolymph (seeSupplementary Video 1) from larvae of the following genotypes:ywF; tub>dmyc>gal4, TyrRS-HA(TyrRS-HA) andyw(WT). Tubulin is used as a negative control to discard contamination from cellular fractions. (e, right panel) Western blot from homogenized larvae of the following genotypes:ywF; tub>dmyc>gal4, UAS-TyrRS-HA(TyrRS-HA);ywF; tub>dmyc>gal4, UAS-TyrRS-HA, UAS-TyrRS-RNAi(TyrRSRNAi) andyw(WT).Western blot of haemolymph from larvae of the following genotype:ywF; tub>dmyc>gal4, TyrRS-HA, BskDN(BskDN), tubulin is used as a loading control. (f) Western blot of the third instar larvae haemolymph 48 h after cell competition clones were induced. GenotypeywF; tub>dmyc>gal4, UAS-LacZ(control),UAS-RNAi TyrRS, UAS-p35, UAS-BskDNorUAS-RNAi Kish.TyrRS cleaved fragments are named according to the molecular weight 51, 46 and 41 kDa. Lipophorin was used as a loading control. (g) Schematic representation of TyrRS including the linker region, MiniTyr domain (41 kDa) that includes the Tyrosine tRNA ligase signature and the C-terminal EMAP domain (17 kDa) including the tRNA-binding domain. (h) Quantification of secreted TyrRS normalized by the loading control Lipophorin (Lip), this ratio from the control is considered as 100%. (i) Cleaved secreted TyrRS/total secreted TyrRS in haemolymph. Control samples are protein extracts from larvae in which cell competition has been induced and loser clones express UAS-LacZ, innocuous for the cell.T-test *P<0.05. s.d. is represented. Figure 3: Loser cells secrete TyrRS under serum deprivation and during cell competition. ( a ) Western blot of cellular fraction and supernatant of Drosophila S2 cells transfected with TyrRS- HA-tagged (C terminus). Cells are cultured with (+) or without (−) serum, as indicated. Anti-HA is used to detect TyrRS-HA expression and anti-tubulin is used as a negative control. ( b , c ) Microscopy images of cultured Drosophila S2 cells with and without serum at 24 h. Sytox Green is used as a marker of cell death. Scale bar, 25 μm. ( d ) Quantifications of total number of cells and dead cells. ( e , left panel) Western blot of haemolymph (see Supplementary Video 1 ) from larvae of the following genotypes: ywF; tub>dmyc>gal4, TyrRS-HA (TyrRS-HA) and yw (WT). Tubulin is used as a negative control to discard contamination from cellular fractions. ( e , right panel) Western blot from homogenized larvae of the following genotypes: ywF; tub>dmyc>gal4, UAS-TyrRS-HA (TyrRS-HA); ywF; tub>dmyc>gal4, UAS-TyrRS-HA, UAS-TyrRS-RNAi (TyrRSRNAi) and yw (WT).Western blot of haemolymph from larvae of the following genotype: ywF; tub>dmyc>gal4, TyrRS-HA, BskDN ( Bsk DN ), tubulin is used as a loading control. ( f ) Western blot of the third instar larvae haemolymph 48 h after cell competition clones were induced. Genotype ywF; tub>dmyc>gal4, UAS-LacZ (control), UAS-RNAi TyrRS, UAS-p35, UAS-Bsk DN or UAS-RNAi Kish. TyrRS cleaved fragments are named according to the molecular weight 51, 46 and 41 kDa. Lipophorin was used as a loading control. ( g ) Schematic representation of TyrRS including the linker region, MiniTyr domain (41 kDa) that includes the Tyrosine tRNA ligase signature and the C-terminal EMAP domain (17 kDa) including the tRNA-binding domain. ( h ) Quantification of secreted TyrRS normalized by the loading control Lipophorin (Lip), this ratio from the control is considered as 100%. ( i ) Cleaved secreted TyrRS/total secreted TyrRS in haemolymph. Control samples are protein extracts from larvae in which cell competition has been induced and loser clones express UAS-LacZ, innocuous for the cell. T -test * P <0.05. s.d. is represented. Full size image To validate this result, we tested whether TyrRS secreted by loser cells in vivo was present in the haemolymph. We induced super-competition in tub>dmyc>gal4; UAS-TyrRS-HA larvae. At 48 h after the induction of super-competition, haemolymph was extracted ( Supplementary Video 1 ; Supplementary Fig. 1 ) and probed in a western blot with anti-HA antibody. TyrRS-HA protein was found in the haemolymph fraction of larvae with super-competition clones ( Fig. 3e , left panel). To verify that the detected HA signal indeed corresponds to TyrRS, the co-expression of UAS-TyrRS-RNAi causes a reduction in the HA-positive band in homogenized larvae ( Fig. 3e , right panel). As JNK signalling is activated during cell competition [4] , we therefore aimed to determine whether TyrRS secretion requires JNK signalling. Again, we induced super-competition in tub>dmyc>gal4; UAS-TyrRS-HA larvae, but now we co-expressed a dominant-negative version of Basket ( Bsk DN ), which inhibits JNK signalling [29] and apoptosis [30] . TyrRS-HA secretion into the haemolymph was reduced when JNK signalling was blocked ( Fig. 3e , right panel), indicating that TyrRS-HA secretion lies downstream of JNK activation and therefore it is a regulated process during cell competition. To detect endogenous TyrRS secretion and cleavage upon cell competition, western blots were done with anti-TyrRS antibody (Covalab) using Lipophorin [26] as a loading control. Third instar larvae haemolymph was extracted 48 h after super-competition (tub>dMyc>gal4) was induced (see Supplementary Fig. 1 and Methods). Full-length (TyrRS) protein as well as TyrRS cleaved fragments (TyrRS51, 46 and 41) were detected ( Fig. 3f ). To determine the pathways involved in TyrRS secretion and cleavage, the following modifications were done in loser cells exposed to super-competition: (1)TyrRS or Kish RNAi-mediated knockdown reduced the amount of total secreted protein ( Fig. 3f,h ), consistent with previous results. (2) Overexpression of p35, an apoptotic inhibitor [31] , increased TyrRS secretion in the haemolymph ( Fig. 3f,h ), which might be due to an increased number of loser cells that do not die but keep secreting the protein. (3) Finally, co-expression of a dominant-negative Basket mutant ( Bsk DN ) that inhibits JNK signalling [29] reduced TyrRS in the haemolymph ( Fig. 3f,h ), indicating that JNK activation is necessary for TyrRS secretion. From these experiments, we conclude that TyrRS secretion is a regulated process during cell competition that does not require caspase activity but rather is secreted by loser cells through a JNK and Kish -dependent mechanism. Secreted TyrRS cleavage is JNK and apoptosis dependent Secreted mammalian TyrRS is cleaved into two fragments that act as distinct cytokines. The enzyme is secreted under apoptotic conditions in the culture media where it is cleaved by proteases into an N-terminal fragment (MiniTyrRS) that harbours the catalytic site and functions as an interleukin-8-like cytokine, and into a C-terminal fragment (EMAPII-like domain) with monocyte and leukocyte chemotaxis activity [25] , [32] , [33] , [34] . Alignment of human TyrRS and its Drosophila homologous protein revealed 80% of similarity ( Supplementary Fig. 3A ). Western blots with haemolymph extracts after cell competition showed that secreted TyrRS is cleaved ( Fig. 3f,i ). TyrRS cleavage is prevented if JNK signalling (bskDN) or apoptosis are blocked. Altogether, our results indicate that in flies, just like in humans, TyrRS cleavage is induced by apoptotic loser cells in a JNK-dependent manner. Matrix metalloproteinase Mmp2 cleaves TyrRS in loser cells Human TyrRS has been proposed to generate MiniTyrRS and EMAPII fragments by two different mechanisms: proteolytic cleavage [25] and alternative splicing [35] . To test the proteolytic hypothesis, we used transgenic flies expressing TyrRS-HA that cannot be alternatively spliced. To determine whether TyrRS-HA can be proteolitically cleaved, we performed western blot experiments with protein extracts of flies expressing TyrRS-HA. Anti-HA antibody visualized two bands, one representing the full-length TyrRS-HA protein and another one representing the 51 Kd HA-tagged C-terminal fragment, TyrRS51 (arrowheads in Fig. 4a ). This result suggests that TyrRS in Drosophila is cleaved in vivo . 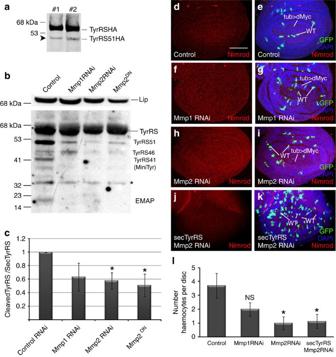Figure 4: Secreted TyrRS is cleaved by matrix metalloproteinase 2 during cell competition. (a) Western blot with protein extracts of larvae expressing TyrRS-HA-tagged protein incubated with the anti-HA antibody, full-length TyrRS-HA is detected and a smaller fragment product of proteolytic cleavage (TyrRS51-HA) are detected. (b) Western blot of the third instar larvae haemolymph 48 h after cell competition clones were induced. GenotypeywF; tub>dmyc>gal4, UAS-LacZ(control),UAS-RNAi Mmp1, UAS-RNAi Mmp2, UAS-Mmp2DN. Lip-Lipophorin, TyrRS-full-length TyrRS, TyrRS 52, 46 and 41 kDa are cleaved fragments of TyrRS, *Unspecific band, 17-kDa fragments corresponds to EMAP and/or MiniTyr molecular weight. Lipophorin was used as a loading control. (c) Quantification of total secreted TyrRS/total TyrRS protein normalized by the loading control (Lipophorin) in haemolymph of the third instar larvae 48 ACI; experiments represent the average of three independent experiments. * is statistically significant,T-testP<0.05; s.d. is represented. (d–i) Haemocyte staining (Nimrod, red) in wing imaginal discs with clones ofwtloser cells (green, GFP) under cell competition 48 h after heat shock (ACI). (d,e) Control loser cells expressing LacZ, (f,g) loser cells expressingMmp1 RNAiand (h,i) loser cells expressingMmp2 RNAi. (j,k) Haemocyte staining (Nimrod, red) in wing imaginal discs with clones of cells (green, GFP) expressing secreted TyrRS (secTyrRS) andMmp2 RNAi 48 h after heat shock (ACI). Nuclei are marked in blue (DAPI). (l) Number of haemocytes per disc quantification (n=10 discs). * is statistically significant,T-testP<0.05; s.d. is represented. Scale bar, 50 μm. DAPI, 4,6-diamidino-2-phenylindole; NS, not significant. Figure 4: Secreted TyrRS is cleaved by matrix metalloproteinase 2 during cell competition. ( a ) Western blot with protein extracts of larvae expressing TyrRS-HA-tagged protein incubated with the anti-HA antibody, full-length TyrRS-HA is detected and a smaller fragment product of proteolytic cleavage (TyrRS51-HA) are detected. ( b ) Western blot of the third instar larvae haemolymph 48 h after cell competition clones were induced. Genotype ywF; tub>dmyc>gal4, UAS-LacZ (control), UAS-RNAi Mmp1, UAS-RNAi Mmp2, UAS-Mmp2 DN . Lip-Lipophorin, TyrRS-full-length TyrRS, TyrRS 52, 46 and 41 kDa are cleaved fragments of TyrRS, *Unspecific band, 17-kDa fragments corresponds to EMAP and/or MiniTyr molecular weight. Lipophorin was used as a loading control. ( c ) Quantification of total secreted TyrRS/total TyrRS protein normalized by the loading control (Lipophorin) in haemolymph of the third instar larvae 48 ACI; experiments represent the average of three independent experiments. * is statistically significant, T -test P <0.05; s.d. is represented. ( d – i ) Haemocyte staining (Nimrod, red) in wing imaginal discs with clones of wt loser cells (green, GFP) under cell competition 48 h after heat shock (ACI). ( d , e ) Control loser cells expressing LacZ, ( f , g ) loser cells expressing Mmp1 RNAi and ( h , i ) loser cells expressing Mmp2 RNAi . ( j , k ) Haemocyte staining (Nimrod, red) in wing imaginal discs with clones of cells (green, GFP) expressing secreted TyrRS (secTyrRS) and Mmp2 RNA i 48 h after heat shock (ACI). Nuclei are marked in blue (DAPI). ( l ) Number of haemocytes per disc quantification ( n =10 discs). * is statistically significant, T -test P <0.05; s.d. is represented. Scale bar, 50 μm. DAPI, 4,6-diamidino-2-phenylindole; NS, not significant. Full size image To test the second hypothesis, namely the alternative splicing, we performed reverse transcription–PCR experiments with specific TyrRS primers; nevertheless, we did not detect any spliced messenger RNA. Even though, we cannot discard this hypothesis, a series of multiplex PCRs, deep-sequencing analysis, in vitro translation of the splice variants detected as well as mass spectrometry analysis of the translated proteins would be required, all of which are beyond the scope of this study. On these grounds, we have decided to focus on the first hypothesis although accepting that alternative splicing may well be playing a role too. To further investigate the proteolytic hypothesis, we evaluated the contribution of Mmp in the cleavage of TyrRS. There are two Mmp orthologues in Drosophila , Mmp1 and Mmp2 , and both genes are transcriptionally regulated by JNK [36] , [37] . Mmp are extracellular endopeptidases involved in the processing of extracellular matrix proteins, the cleavage of cell surface receptors, the release of apoptotic ligands and the chemokine/cytokine regulation [38] , [39] , [40] , [41] , [42] . To determine whether the effect of JNK signalling in TyrRS cleavage depends on Mmps, we silenced Mmp1 or Mmp2 transcripts in loser cells during cell competition. Western blot experiments of third instar larvae protein extracts 48 h ACI were hybridized with anti-TyrRS and lipophorin antibodies ( Fig. 4b ) and revealed that the knockdown of Mmp1 did not significantly reduce the cleavage of TyrRS to Tyr51, 46, 41 (MiniTyr) and EMAP (17 Kd) fragments. On the other hand, RNAi-mediated knockdown of Mmp2 or forced expression of Mmp2 DN prevented the cleavage of TyrRS ( Fig. 4b,c ). To determine whether Mmps cleave TyrRS during haemocyte recruitment, we stained the haemocytes with a haemocyte marker Nimrod [43] in the wing imaginal discs during cell competition after silencing the expression of Mmp1 or Mmp2 in loser cells ( Fig. 4d–i ). Our results indicate that the number and size of loser cell clones was unchanged in these wing imaginal discs; however, there was a significant reduction in haemocyte number per wing disc upon Mmp2 RNAi- mediated silencing in loser cells ( Fig. 4l ). On the contrary, the number of haemocytes per disc upon RNAi-mediated knockdown of Mmp1 in loser cells was unaffected, though a slight but statistically insignificant reduction was observed. Finally, to further define the role of Mmp2 in the recruitment of haemocytes upon TyrRS secretion, we generated WT clones of cell in a WT background (without cell competition). Expression of a secreted form of TyrRS (see Methods) together with RNAi-mediated silencing of Mmp2 abolished haemocyte recruitment. Altogether, our data suggest that secreted TyrRS is cleaved by Mmp2, and that these extracellular TyrRS fragments recruit haemocytes to the site of cell competition. Secreted TyrRS acts as a chemoattractive cue for haemocytes It has been previously shown that cleaved extracellular human TyrRS fragments (EMAPII) attract macrophages, which then remove the apoptotic cells [25] . To analyse the activity of TyrRS as a chemoattractant, we generated a constitutively secreted TyrRS (secTyrRS) by fusing TyrRS with a signal peptide (see Methods), and performed a chemotaxis assay ( Supplementary Fig. 4 ; Fig. 5a,b ). In all experiments, the upper compartment of the chemotaxis chamber contained S2 cells marked with CellTracker Red. The lower compartment contained either S2 cells transfected with act-gal4 plasmid (Control) or act-gal4 UAS-secTyrRS (secTyrRS). After 48 h of incubation, we counted the number of red cells on the basal side of the transwell membrane in six independent experiments. Our results indicate that a significant number of Red S2 cells migrated towards the lower chamber when it contained the secTyrRS -transfected cells but not the control cells ( Fig. 5a–c ; Supplementary Video 2 ; Supplementary Video 3 ), suggesting that secTyrRS has chemoattractant capacity in Drosophila S2 cells. 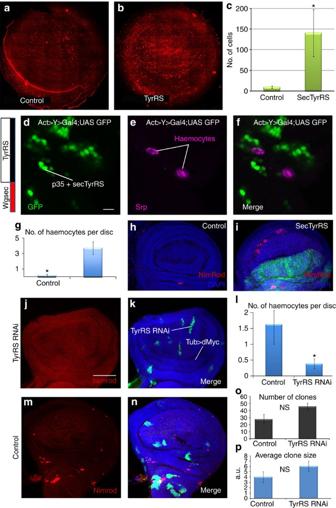Figure 5: Secreted TyrRS acts as a ‘find me’ signal for haemocytes. (a–c) S2 cells transfected withact-gal4plasmid alone (Control) oract-gal4 UAS-secTyrRS(secTyrRS), were plated on the lower compartment of the chemotaxis chamber. On the upper membrane of the transwell, S2 cells (red) were marked with CellTracker Red (Life Technologies) and incubated for 48 h. The number of cells that were attracted to the basal side of the transwell membrane was counted in six independent experiments.T-test *P<0.05. The secreted form ofDrosophilaTyrRS (secTyrRS) induces the attraction of haemocytes (Serpent, magenta) when is overexpressed in wild-type clones (GFP, green). (d–f). Scale, bar 10 μm. The same phenotype is achieved whensecTyrRSorTyrRSis expressed in the dorsal compartment (apterous-gal4).In all, 24 wing discs were measured for each genotype (g–i).T-test *P<0.05. Knockdown of TyrRS in loser cells (GFP) (j,k) or control (LacZ) cells (m,n) 48 h after induction of super-competition. Scale bar 25 μm. Nuclei are marked in blue (4,6-diamidino-2-phenylindole (DAPI)). (l) Quantification of the number of haemocytes in discs with super-competition clones, 21 wing discs were measured for each genotype. Quantification of the number of clones (o) or size of the clones (p) during cell competition 48 ACI between LacZ expressing clones (LacZ) andTyrRS RNAi-expressing clones.T-test *P<0.05, NS, non significant;n=10 discs. Figure 5: Secreted TyrRS acts as a ‘find me’ signal for haemocytes. ( a – c ) S2 cells transfected with act-gal4 plasmid alone (Control) or act-gal4 UAS-secTyrRS (secTyrRS), were plated on the lower compartment of the chemotaxis chamber. On the upper membrane of the transwell, S2 cells (red) were marked with CellTracker Red (Life Technologies) and incubated for 48 h. The number of cells that were attracted to the basal side of the transwell membrane was counted in six independent experiments. T -test * P <0.05. The secreted form of Drosophila TyrRS (secTyrRS) induces the attraction of haemocytes (Serpent, magenta) when is overexpressed in wild-type clones (GFP, green). ( d – f ). Scale, bar 10 μm. The same phenotype is achieved when secTyrRS or TyrRS is expressed in the dorsal compartment ( apterous-gal4). In all, 24 wing discs were measured for each genotype ( g – i ). T -test * P <0.05. Knockdown of TyrRS in loser cells (GFP) ( j , k ) or control (LacZ) cells ( m , n ) 48 h after induction of super-competition. Scale bar 25 μm. Nuclei are marked in blue (4,6-diamidino-2-phenylindole (DAPI)). ( l ) Quantification of the number of haemocytes in discs with super-competition clones, 21 wing discs were measured for each genotype. Quantification of the number of clones ( o ) or size of the clones ( p ) during cell competition 48 ACI between LacZ expressing clones (LacZ) and TyrRS RNAi -expressing clones. T -test * P <0.05, NS, non significant; n =10 discs. Full size image We then studied the mechanism of TyrRS function in vivo by using transgenic flies expressing the constitutively secreted TyrRS (secTyrRS). To test whether secTyrRS was sufficient to act as a haemocyte chemoattractant, we co-expressed UAS- secTyrRS with UAS-p35 to prevent apoptosis in the wing imaginal discs. Staining against the haemocyte marker Serpent showed that secTyrRS expression in wt clones was sufficient to attract haemocytes in the absence of competition ( Fig. 5d–f ). Moreover, we examined the recruitment abilities of secTyrRS by overexpressing it in the dorsal compartment of the wing discs via the apterous-gal4 driver. Again, haemocyte recruitment, visualized by Nimrod staining, was observed when secTyrRS was expressed in the dorsal (apterous) compartment, compared with a control situation ( Fig. 5g–i ; quantified in Fig. 5g ). Finally, to determine whether TyrRS is necessary for haemocyte recruitment during super-competition, we silenced TyrRS gene expression in loser cells, which inhibited haemocyte recruitment ( Fig. 5j–n ). The number and size of loser cell clones upon RNAi-mediated TyrRS silencing was not significantly different from the control samples, indicating that the observed difference in haemocyte recruitment was not affected by these parameters ( Fig. 5o,p ). Taken together, these results show that the presence of secreted TyrRS protein is required and sufficient to recruit circulating haemocytes towards TyrRS-secreting cells. Secreted EMAP act as a chemoattractant for haemocytes Next, we asked which of the cleaved fragments of TyrRS is capable of attracting haemocytes. It has been described that human TyrRS C-Terminal fragment (EMAPII-like domain) has chemoattractant activity for monocytes and leukocytes [25] , [32] , [34] . To address this point, we generated transgenic UAS flies with cytoplasmic and secreted versions of Drosophila TyrRS, MiniTyr (Tyrosine tRNA ligase+linker domains) (41 Kd) and EMAP (17 Kd) (see Methods). To verify that secreted transgenic forms are indeed secreted and properly cleaved, we performed western blots using haemolymph from larvae expressing each construct under the control of engrailed promoter (en-Gal4) ( Supplementary Fig. 5 ). Next, we expressed each of these constructs under the control of apterous-gal4 promoter in the wing imaginal disc (marked in green, UAS-GFP) and stained for haemocytes with Nimrod antibody. As previously shown ( Fig. 5i ), TyrRS has to be secreted to induce haemocyte recruitment ( Fig. 6a–d,m ). Cellular MiniTyr and EMAP fragments did not cause haemocyte recruitment ( Fig. 6e,g,i,k,m ). However, whereas the secretion of MiniTyr in the apterous domain was lethal, secreted EMAP showed haemocyte recruitment activity comparable to that of the secreted TyrRS ( Fig. 6b,j,m ). To further investigate this phenomenon, we generated WT clones in imaginal discs and visualized the apoptotic cells by Caspase-3 staining ( Supplementary Fig. 6 ). We found that both secreted TyrRS and MiniTyr induce apoptosis, as shown by red Caspase-3 staining of the GFP-positive cells. Collectively, these results indicate that EMAP once released, is capable of recruiting haemocytes to the sites where apoptotic cells are localized. 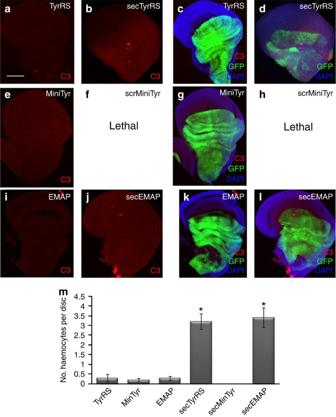Figure 6: Secreted TyrRS or EMAP domain chemo-attracts haemocytes. (a–l) Active Caspase-3 staining (red) in wing imaginal discs of third instar larvae that express TyrRS (a,c), secreted TyrRS (b,d), MiniTyr (e,g), secreted MiniTyr (f,hlethal), EMAP (i,k) or secreted EMAP (j,l) underapterous-gal4enhancer (green, GFP marked). Nuclei are marked in blue (DAPI). (m) Number of haemocytes per disc quantification. * is statistically significant,T-testP<0.05; s.d. is represented.n=10 disc. Scale bar, 25 μm. DAPI, 4,6-diamidino-2-phenylindole. Figure 6: Secreted TyrRS or EMAP domain chemo-attracts haemocytes. ( a – l ) Active Caspase-3 staining (red) in wing imaginal discs of third instar larvae that express TyrRS ( a , c ), secreted TyrRS ( b , d ), MiniTyr ( e , g ), secreted MiniTyr ( f , h lethal), EMAP ( i , k ) or secreted EMAP ( j , l ) under apterous-gal4 enhancer (green, GFP marked). Nuclei are marked in blue (DAPI). ( m ) Number of haemocytes per disc quantification. * is statistically significant, T -test P <0.05; s.d. is represented. n =10 disc. Scale bar, 25 μm. DAPI, 4,6-diamidino-2-phenylindole. Full size image TyrRS triggers PI3K activation in haemocytes To further characterize the mechanism of haemocyte recruitment, we asked which changes TyrRS could provoke in circulating haemocytes. Different studies have shown that the phosphoinositides PtdINS(3,4,5)P3 (PIP3) and PtdIns(3,4)P2 (PIP2) are rapidly polarized in cells exposed to a chemoattractant gradient [44] . Phosphoinositide-3 kinases translocate from the cytosol to the membrane at the leading edge of the chemotaxing cell, whereas phosphatase and tensin homologues (PTEN) relocate to the rear. In Drosophila , there is only one class of PI3K, named Dp110, that has been shown to have a role in cell growth and haemocyte migration [45] , [46] . We therefore studied the connection between PI3K and TyrRS-mediated haemocyte chemotaxis. To do that we performed the haemocyte attraction assay by overexpressing secTyrRS in the dorsal compartment of wing imaginal discs. At the same time, we overexpressed a reporter of PI3K activity that includes the PH domain of PIP (PH-GFP). This reporter causes GFP signal accumulation in the membrane upon PI3K activation [47] . We observed a punctuated GFP signal associated with haemocytes plasma membrane when secTyrRS was expressed in the dorsal compartment of the wing imaginal disc ( apterous-gal4 , GFP) ( Fig. 7d–g ) but not in the control cells expressing beta-galactosidase (LacZ) ( Fig. 7a–c ). This result suggests that TyrRS secretion can activate PI3K in haemocytes. 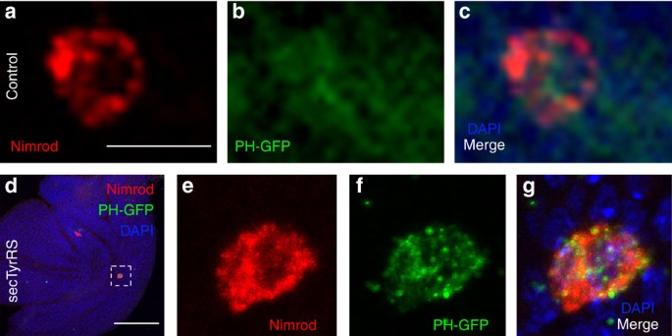Figure 7: TyrRS activates PI3K signalling in haemocytes. Haemocytes (red-NimRod) are recruited after secretedTyrRSexpression in the dorsal compartment, and PI3K signalling (green-PH_GFP) is activated in these haemocytes. PH-GFP is accumulated in the membranes when PI3K signalling is activated (d–g) compared with the control situation expressing beta-galactosidase (LacZ) (a–c). (a–c,e–g) Magnifications of haemocytes in wing imaginal discs of the third instar larvae. Scale bar, 10 μm. (d) Wing imaginal discs of the third instar larvae expressing secretedTyrRSwith recruited haemocytes (white dotted lines). Scale bar, 25 μm. DAPI, 4,6-diamidino-2-phenylindole. Figure 7: TyrRS activates PI3K signalling in haemocytes. Haemocytes (red-NimRod) are recruited after secreted TyrRS expression in the dorsal compartment, and PI3K signalling (green-PH_GFP) is activated in these haemocytes. PH-GFP is accumulated in the membranes when PI3K signalling is activated ( d – g ) compared with the control situation expressing beta-galactosidase (LacZ) ( a – c ). ( a – c , e – g ) Magnifications of haemocytes in wing imaginal discs of the third instar larvae. Scale bar, 10 μm. ( d ) Wing imaginal discs of the third instar larvae expressing secreted TyrRS with recruited haemocytes (white dotted lines). Scale bar, 25 μm. DAPI, 4,6-diamidino-2-phenylindole. Full size image It is well known that chemotaxis guides the macrophages towards apoptotic cells in mammals [48] , [49] . This process is regulated by molecules released from the dying cells [50] . First, the long-range chemotactic signals (‘find me’ signals) form concentration gradients that attract macrophages towards the source [51] , [52] , [53] , [54] , [55] . Second, the short range signals (‘eat me’ signals) that are present at the membrane of the dying cells enable the contact between the macrophage and the target [56] , leading to engulfment of the apoptotic cells [57] . However, it is possible that chemotaxis of mammalian macrophages may be an evolutionary adaptation of bigger organisms that enables them to solve the problem of finding small targets, such as dying cells, in a large internal volume. In animals with a small body size similar to Drosophila [58] , where the internal environment is several times smaller, chemotaxis may be unnecessary and the circulating macrophages (haemocytes in Drosophila ) may arrive unguided at the sites where the ‘eat me’ signals are present. Indeed, despite extensive research in apoptosis and phagocytosis [59] , [60] , no apoptosis-dedicated attractant for haemocytes has been described in Drosophila . Only molecules that act as ‘eat me signals’ [61] , [62] have been reported, as well as signalling pathways that stimulate haemocyte proliferation within damaged tissues [63] . Three mechanisms have been shown to direct haemocyte migration in Drosophila embryos: the receptor tyrosine kinase, PVR, controls haemocyte migration during embryogenesis [64] as well as proliferation [65] and survival [66] , during developmental migration [46] . Conversely, PI3K-mediated migration is crucial for haemocytes to sense a chemotactic gradient from a wound, but not for developmental migration [46] , [67] . Finally, hydrogen peroxide (H 2 O 2 ) has been identified as the earliest wound attractant in Drosophila embryos and zebrafish larvae [68] . We have shown that Drosophila haemocytes are recruited towards the basal regions where cell competition is taking place to remove apoptotic cells [10] . Other authors have reported that winner cells engulf the M/+ loser in the apical region of the epithelium through Draper [9] , [11] . With that in mind, we cannot fully exclude that winner cells can engulf a few loser cells in the apical zone of the imaginal discs; however, we have never observed such an event. We found that haemocytes engulf >95% of the loser cells [10] , and that the engulfment step does not play a causal role to induce death in losers, but is rather required to clear apoptotic debris [10] . Pastor-Pareja et al. have shown that expression of the unpaired cytokines 1, 2 and 3 ( upd 1 , 2 and 3 ) induce haemocyte proliferation in response to JNK activation in scribbled mutant tumours or damaged tissue [63] . They proposed that haemocytes could reach the damaged area by a random process, however, our results support a scenario in which loser cells require JNK signalling to actively secrete TyrRS, which is then cleaved in the extracellular space and acting as a signal to attract haemocytes during cell competition ( Fig. 8 ). The chemoattractant function of the secreted TyrRS appears to be conserved between flies and humans. It is tempting to speculate that such a signal may be important for animals with a coelom fluid-filled cavity, to allow the scavenger cells to navigate the evolutionary innovation of the internal medium. 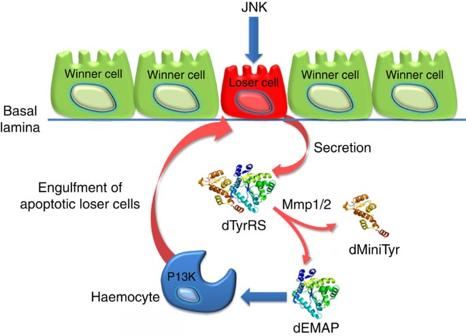Figure 8: TyrRS secretion and cleavage model. During cell competition, winner cells (green) induce the elimination of loser cells (red) by apoptosis. Loser cells, via JNK, secrete TyrRS that is cleaved by Mmp1/2 to generate MiniTyr and EMAP fragments. The PI3K pathway is activated in haemocytes that are recruited to the region of cell competition by EMAP to engulf apoptotic loser cells. Figure 8: TyrRS secretion and cleavage model. During cell competition, winner cells (green) induce the elimination of loser cells (red) by apoptosis. Loser cells, via JNK, secrete TyrRS that is cleaved by Mmp1/2 to generate MiniTyr and EMAP fragments. The PI3K pathway is activated in haemocytes that are recruited to the region of cell competition by EMAP to engulf apoptotic loser cells. Full size image TyrRS, similar to other AARS, is part of the protein synthesis machinery. In particular, TyrRS is responsible for catalysing the binding reaction between tyrosine and its corresponding tRNA. Similarly, and like other AARS, TyrRS has evolved and incorporated new functional domains, such as EMAPII domain, which is conserved from insects to humans (reviewed in ref. 69 ). We have shown that Drosophila TyrRS is secreted under apoptotic conditions similarly to what happens in human cells [25] . The secreted TyrRS is then cleaved by metalloproteinases producing MiniTyr and EMAP fragments. Our results suggest that the latter fragment acts as a haemocyte chemoattractant. Haemocytes, activate PI3K in response to secreted TyrRS and migrate towards the apoptotic cells. We also show that TyrRS secretion is controlled by JNK signalling and regulated by different components of the secretory pathway such as kish and gryzun. Although we have established kish and gryzun dependence, the mechanisms for secretion is clearly due to a non-classical pathway that is currently unknown. It has been previously suggested that secretion of a core component of the translational machinery would be expected to arrest translation and thereby accelerate apoptosis [25] . Both TyrRS- and MiniTyr-induced-secretion trigger cell apoptosis, whereas EMAP secretion does not. This result could be a consequence of the expression of the artificially secreted proteins such as secMiniTyr, as under normal conditions TyrRS is first secreted and then cleaved to generate MiniTyr and EMAP fragments. Whether the MiniTyr fragment triggers apoptosis as a killing signal acting intracellularly or extracellularly is presently still unknown. It is unknown whether TyrRS secretion is a general mechanism for haemocyte recruitment or if it is specific for apoptotic cells resulting from cell competition. It is also unknown which receptor(s) recognize extracellular TyrRS to activate PI3K in haemocytes. Further work will be required to clarify these points. In summary, we show that JNK signalling- and Kish- mediated secretion of TyrRS from the dying loser cells transform an enzyme into a signalling molecule that acts as a haemocyte chemoattractant. Subsequently, haemocytes migrate along TyrRS gradients to localize and engulf apoptotic cells. TyrRS cloning recombination clones and haemocyte experiments The fly stocks were obtained from the Bloomington Stock Center, except where indicated. For haemolymph analysis, TyrRS complementary DNA (cDNA) was cloned into EcoRI and XhoI restriction sites of pUAST in frame with the C-terminal haemagglutinin tag (sequence: 5-′TACCCATACGATGTTCCAGATTACGCT-3′) to obtain TyrRS-HA. To study the secretion of TyrRS-HA in super-competition, the recombinant stock ywhs-FLP; tub>dmyc>gal4, UAS-TyrRS-HA/Cyo; UAS-GFP/TM6B was generated and crossed with UAS- Kish RNAi (from VDRC GD: no. 40884), UAS- Gryzun RNAi (from VDRC KK: no. 105660) or UAS-LacZ males. The larvae were subjected to a 15-min heat shock at 37 °C and analysed at 48 h ACI by immunofluorescence. For haemolymph analysis of endogenous TyrRS, females of the genotype ywhs-FLP; tub>dmyc>gal4 were crossed with UAS-LacZ males and yw flies were used as a negative control. The larvae were subjected to a 15-min heat shock at 37 °C and analysed at 48 h ACI by extracting the haemolymph and analysing by western blot. To study the relation between TyrRS-HA secretion and JNK pathway, females of the genotype ywhs-FLP; tub>dmyc>gal4, TyrRS-HA/Cyo; UAS-GFP/TM6B were crossed with UAS-BskDN or UAS-TyrRS RNAi (from GD: no. v40541) males. To study the endogenous TyrRS, females of the genotype ywhs-FLP; tub>dmyc>gal4 were crossed with UAS-TyrRS RNAi (from GD: no. v40541) or UAS-LacZ males. Larvae were subjected to 15-min heat shock at 37 °C and analysed at 48 h ACI by extracting the haemolymph and examining by western blot. Finally, to study TyrRS secretion blocking cell death by p35, females of the genotype ywh-FLP; UAS-p35/”; act>y+>gal4, UAS-GFP/TM6B were crossed to UAS-TyrRS-HA/” males. Larvae were subjected to 10-min heat shock at 37 °C and analysed at 48 h ACI by western blot. Homogenized larvae where TyrRS-HA was ubiquitously expressed were used as a positive control for HA staining and yw flies were used as a negative control. To study the implication of the metalloproteinases Mmp1 and Mmp2 in TyrRS cleavage, females of the genotype ywhs-FLP; tub>dmyc>gal4 were crossed with UAS-Mmp1 RNAi (from VDRC KK: no. 101505), UAS-Mmp2 RNAi (from VDRC KK: no. 107888) or UAS-LacZ males. For haemocyte attraction experiments, TyrRS cDNA was cloned into EcoRI and XhoI restriction sites of pUAST in frame with the N-terminal Wingless secretion peptide (sequence: 5′-ATGGATATCAGCTATATCTTCGTCATCTG CCTGATGGCCCTGTGCAGCGGC-3′) to obtain UAS-Sec TyrRS transgenic flies. To block apoptosis females of genotype ywhs-FLP; UAS-p35/”; act>y+>gal4, UAS-GFP/TM6B were crossed with UAS-Sec TyrRS males. The larvae were heat shocked for 10 min at 37 °C and dissected at 48 h ACI. In the case of apterous crosses, females of the genotype w; apgal4 UAS-GFP/Cyo were crossed with UAS-Sec TyrRS males. Larvae were dissected at the third larval instar. To study the implication of TyrRS in the recruitment of haemocytes, females of the genotype ywhs-FLP; tub>dmyc>gal4 were crossed with UAS-TyrRS RNAi (from GD: no. v40541) or UAS-LacZ males. To study the cytokine activities of TyrRS and its fragments, five transgenic lines were generated: – UAS-TyrRS ; TyrRS cDNA was cloned into EcoRI and XhoI restriction sites of pUAST. – UAS-MiniTyr ; Drosophila MiniTyr cDNA (located at the N-terminal of TyrRS, according to human MiniTyr homologue sequence) was cloned into EcoRI and XhoI restriction sites of pUAST. MiniTyr sequence (molecular weight 41 kDa) 5′-ATGGTCGGAATAACGCCCGCAGAGAAGAAAGCGCTGATAACGCGCAATCTGCAGGAGACGCTCGGCGATGACAAGCTGACCAAGATCCTGGCGGAGCGCGATCTAAAGATCTACTGGGGAACGGCGACGACGGGCAAGCCACATGTCGCCTATTTCGTGCCCATGTCGAAGATTGCCGATTTCCTGAAGGCAGGATGCGAAGTGACCATCCTGTTCGCCGATCTCCACGCCTATCTGGACAACATGAAGGCACCGTGGTCTCTCCTGGAGCTGCGAACCAAGTACTACGAACAGGTCATCAAGGCCATGTTGAGCTCCATCGGCGTTCCGCTGGAGAAACTGAAGTTCGTCAAGGGCAGCGACTATCAGCTGTCCAAGGAGTACACCCTGGATGTATACAAGCTCAGCTCCGTGGTCACGCAACACGATGCCAAGAAGGCGGGCGCAGAGGTGGTCAAACAGTGGAGTACCCACTGCTCTCCGGTTTGCTTTATCCTGGTCTGCAGGCTCTGGACGAGGAGTACCTCAAGGTGGACGCACAATTCGGTGGCGTGGATCAGCGCAAGATCTTTACCTTCTCAGAGAAGTATCTGCCGCAGTTGGGCTACGAAAAGCGCATTCACTTCATGAATCCCATGGTTCCCGGCTTGGCTGGTGGCAAGATGTCCTCTTCCGAGGAGGACTCAAAGATCGATCTTCTGGACTCCCCGGCCAACGTGAAGAAGAAGCTGAAGAAGGCTTTCTGTGAGCCGGGAAACATTGCCGACAACGGCCTGCTGTCCTTCGTGAAGCACGTCCTGTTCTCGCTGTTCAAGGAAGGCGAAGGCTTCGAGGTTAACCGCGAGGCGGAGCATGGCGGCGATGTTACCTTCCTGAAATACGAGGATCTGGAGAAGTACTACGCGGAGGACAAACTGCACCCGGGTGACCTGAAGGCCACCGTGGAGAAGTACATCAACCGACTGCTAGATCCCATTCGAAAGGCCTTTGAAAACCCAGAACTGCAAAAACTGAGTGCTGCTGCTTATCCACCGCCTGCCAAGGTGAAGGCAGGAGCTGCTCCCGCTGCTGGAGCTGACGAAGATGCACCC-3′. – UAS-EMAP ; Drosophila EMAP cDNA (located at the C-terminal of TyrRS, according to the human EMAP homologue sequence) was cloned into EcoRI and XhoI restriction sites of pUAST. EMAP sequence (estimated molecular weight: 17 kDa) 5′-CATCGCCTGGATATCCGCGTGGGCAAGGTCGTCGAGGTGGCCCGTCATCCAGATGCCGATACTCTATATGTGCTGAAGATAGACTTGGCTGAGGCGCAACCCAGAACGATTATTAGTGGCCTGGTGAAGTTTGTCACCGAGGAGGAGCTGAACCAGCGATTGGTGGCGGTTCTTTGCAACCTGAAGCCGTCCAAGATGCGCGGCATCTTGTCCGAGGGCATGGTTCTGTGCACCTCCAACGCTGACCACACGGTGGTGGAGCCTATTGTGCTGCCAGCCACTGCTACTGCTGGCAGTCGCCTCTCCTTCGAGGGATTCAGTGGCACGCCCGATGAGCAGCTTAATCCCAAGAAGAAGGTGTGGGAGAAACTCTCCGCCGACTTCAAGACGAACAGCGATGGACTGGCCGTGTGGAAGGACAACTTCCTGCTGACGCCCGAGGGCGAAAAGCTTTCCAGCAAGCTGGCCAACTGCTCCATTAAATAA-3′. – UAS-sec MiniTyr ; Drosophila MiniTyr cDNA in frame with the N-terminal Wingless secretion peptide was cloned into EcoRI and XhoI restriction sites of pUAST. – UAS-sec EMAP ; Drosophila EMAP cDNA in frame with the N-terminal Wingless secretion peptide was cloned into EcoRI and XhoI restriction sites of pUAST. To study their cytokine abilities, females of the genotype w; apgal4 UAS-GFP/Cyo; were crossed with UAS-TyrRS, UAS-sec TyrRS/”, UAS-MiniTyr, UAS-sec MiniTyr, UAS-EMAP or UAS-sec EMAP males. Larvae were dissected at the third larval instar. Finally, to analyse PI3K activation in haemocytes, females of the genotype en-Gal4; PH-GFP were crossed with UAS-Sec TyrRS or UAS-LacZ males. Larvae were dissected at the third larval instar. All crosses were maintained at 25 °C unless other indication. Haemolymph extraction and preparation All solutions and tools used were sterile. Haemolymph extraction was performed with a TranferMan NK 2 micromanipulator dotted with a CellTram Air. For injection, TransferTips-F glass capillaries (ICSI) broken until having 40-m inner diameter tips were used. Larvae of the different genotypes were grouped together in a dry-ice-cooled adaptor for a Leica DMI-6000 inverted microscope, equipped with a Hamamatsu CCD camera and imaged with LAS AF software from Leica. Their haemolymph was loaded into individual capillaries using the CellTram Air (see Supplementary Video 1 ; Supplementary Fig. 1 ) and transferred to an Eppendorf tube with 10 μl of cooled appropriate buffer (PBS/NaCl 150 mM/ Triton 1% and Protease Inhibitors Cocktail (Roche)). Samples were centrifuged at 10,000 r.p.m. for 10 min to eliminate suspension cells. Finally, the samples were analysed by western blot. Cell culture and transactivation assays The plasmid actα1>gal4 (gift of K. Basler) was used in the transfections to activate the UAS constructs. TyrRS cDNA was cloned into EcoRI and XhoI restriction sites of pUAST in frame with a C-terminal HA epitope with the following sequence: 5′-TACCCATACGATGTTCCAGATTACGCT-3′. The pUASTGFP vector was used as control. In all, 1.5 × 10 6 S2 cells were transfected with SuperFect (Qiagen) using 0.2 μg DNA from each plasmid, efficiency of transfection was around 40%. Cells were treated with PBS/NaCl 150 mM/Triton 1% buffer to extract proteins. For serum deprivation experiments, cells were cultured in Schneider’s medium (Sigma) 10% serum fetal bovine and antibiotics (penicillin and streptomycin, 50 IU ml −1 ) in 12-well plates for 24 h. Medium was substituted with serum-free medium (Grace’s insect media; Lonza) in half of the wells or normal medium in the other half. Cells were maintained for further 24 h. Then, supernatant and the cell pellet of both conditions were recovered at 6 and 24 h. Western blotting For western blots, we used NuPAGE Bis-Tris Gels 4–12% (Invitrogen), and the following primary antibodies: rat anti-HA antibody (1:2,000, Roche), mouse anti-tubulin (1:10,000, Sigma), rabbit anti- Drosophila melanogaster TyrRS (1:500, Covalab) and rabbit anti-lipophorin (1/10,000, gift from James Culi). Original western blot images are included in Supplementary Fig. 7 . Chemotaxis experiments Drosophila S2 cells were plated in the lower compartment of a chemotaxis chamber (6.5 mm Transwell with 5.0 μm Pore Polycarbonate Membrane Insert, Sterile, Corning Life Sciences), and were either transfected with act-gal4 plasmid (control situation) or act-gal4 and UAS-secTyrRS (chemotactic situation). Then, S2 cells stained with Cell TrackerTM Red (CMTPX, Life Technologies) were added to the upper compartment and incubated at room temperature. Cell migration was monitored for 24 h at a rate of one frame every 10 min. After 48 h of incubation, migrating cells were fixed and counted under a fluorescent microscope. Immunohistochemistry The following primary antibodies were used: mouse anti-β galactosidase (1:500, Sigma), rabbit anti- Drosophila melanogaster TyrRS (1:500, Covalab), mouse anti-Serpent (1:1,000) (gift from Pastor-Pareja), rat anti-HA (1:500, Roche), mouse anti-NimRod (1:500, gift from Eva Kurucz) and rabbit anti-Caspase 3 (1:500, Cell Signaling). The following secondary antibodies were used: Alexa Fluor R donkey anti-mouse 647 (1:250, Invitrogen), Alexa Fluor R goat anti-rat 546 (1:250, Invitrogen), Alexa Fluor R goat anti-rat 568 (1:250, Invitrogen). All images were obtained with a LEICA TCS-SP2-AOBS. Fly eyes imaging Adult flies were anaesthetized (CO 2 ) and images were captured using a Leica M165FC microscope and a DC300 camera. Mitotic recombination clones and haemolymph controls The fly stocks used were obtained from the Bloomington Stock Center except where indicated. To analyse the implication of kish in TyrRS secretion during super-competition, females of the genotype ywhs-FLP; tub>dmyc>gal4 were crossed with UAS-gryzun RNAi (from GD: no. 40884), UAS-yellow RNAi (from KK: no. 106068) or UAS-LacZ males. Larvae were subjected to heat shock for 15 min at 37 °C and analysed at 48 h ACI by extracting the haemolymph and analysing by western blot. To study the effect of kish in wild-type clones, females of genotype ywhs-FLP; act>y+>gal4, UAS-GFP/TM6B were crossed with UAS-LacZ or UAS-kish RNAi males. The larvae were heat shocked for 10 min at 37 °C and dissected at 48 h ACI. To analyse the implication of gryzun in TyrRS secretion during super-competition, females of the genotype ywhs-FLP; tub>dmyc>gal4 were crossed with UAS-gryzun RNAi (from GD: no. 41657) or UAS-LacZ males. Larvae were subjected to heat shock for 15 min at 37 °C and analysed at 48 h ACI. To verify the expression of the secreted constructs, haemolymph analysis of endogenous TyrRS was carried out. Females of the genotype w; engrailed-gal4 UAS-GFP/Cyo were crossed with UAS-secTyrRS, UAS-MiniTyr, UAS-secMiniTyr, UAS-EMAP, UAS-secEMAP males and yw flies were used as a negative control. Larvae were analysed by extracting the haemolymph and examining by western blot. Finally, to analyse the apoptotic activity of the different TyrRS fragments in wild-type clones, females of the genotype ywhs-FLP; UAS-p35/”; act>y+>gal4, UAS-GFP/TM6B were crossed with UAS-TyrRS , UAS-SecTyrRS , UAS-MiniTyr , UAS-SecMiniTyr , UAS-EMAP , UAS-SecEMAP or UAS-LacZ males. Larvae were subjected to heat shock for 10 min at 37 °C and analysed at 48 h ACI. For eye phenotype studies, females of the genotype eyeless>gal4 were crossed with UAS-SecTyrRS , UAS-SecMiniTyr , UAS-SecEMAP or UAS-LacZ males. How to cite this article: Casas-Tintó, S. et al. Active JNK-dependent secretion of Drosophila Tyrosyl-tRNA synthetase by loser cells recruits haemocytes during cell competition. Nat. Commun. 6:10022 doi: 10.1038/ncomms10022 (2015).